Shaping colloids for self-assembly The creation of a new material often starts from the design of its constituent building blocks at a smaller scale. From macromolecules to colloidal architectures, to granular systems, the interactions between basic units of matter can dictate the macroscopic behaviour of the resulting engineered material and even regulate its genesis. Information can be imparted to the building units by altering their physical and chemical properties. In particular, the shape of building blocks has a fundamental role at the colloidal scale, as it can govern the self-organization of particles into hierarchical structures and ultimately into the desired material. Herein we report a simple and general approach to generate an entire zoo of new anisotropic colloids. Our method is based on a controlled deformation of multiphase colloidal particles that can be selectively liquified, polymerized, dissolved and functionalized in bulk. We further demonstrate control over the particle functionalization and coating by realizing patchy and Janus colloids. Designing new building blocks of matter with concepts of geometry and shape in mind is giving rise to a generation of new exciting materials [1] , [2] . Shape has a fundamental role in self-assembly as it can regulate particle recognition [3] , determine the density and the structure of particle packings [4] , [5] , [6] , [7] , [8] , and facilitate binding from ligand molecules [9] , [10] . Ideally, patterned surfaces and tailored functionality could act in concert with the shape anisotropy of the building blocks to focus interactions between particles, and could assist, direct or enhance their self-organization [11] . To match the richness and complexity of the self-assembled structures revealed by recent computer-simulation studies, a great deal of work has been devoted to advance synthetic strategies for the fabrication of patchy and anisotropic colloids [12] , [13] , [14] , [15] , [16] , [17] , [18] . Rarely, however, do fabrication techniques integrate design freedom with high particle throughput. To this end, the use of hybrid materials in swelling and emulsification techniques revealed to be particularly successful for fabricating bulk amounts of particles with single or multiple protrusions [19] , [20] , [21] . Here, we propose a versatile strategy to design and mass-produce colloidal building blocks with complex shapes starting from biphasic colloids whose two phases can be selectively and independently polymerized, liquefied and dissolved. In addition, we show that the same synthetic scheme also enables one to selectively functionalize a specific area on the particle surface or a portion of the particle’s body, thus obtaining patchy and Janus colloids in bulk amounts. Synthesis of biphasic colloids Our method comprises three main steps in which biphasic colloids are first synthesized and then reshaped by surface tension during a series of consecutive phase transformations. In the first step, which we refer to as nucleation, aqueous suspensions of biphasic particles are prepared by heterogeneous nucleation of oil droplets in the presence of solid polystyrene (PS) seeds. The oil consists of 3-methacryloxypropyl trimethoxysilane (TPM) oligomers that are generated in situ via a base-catalysed condensation reaction between hydrolysed TPM monomers. The seeds, depending upon their surface charge, can either be fully engulfed in the oil phase or trapped at the oil–water interface. In particular, negatively charged colloids tend to sit at the interface whereas positively charged particles are entirely encapsulated into the oil droplets. This is illustrated in Fig. 1 a showing the heterogeneous nucleation of oil droplets in the presence of, respectively, sulphonated and amine-modified PS particles. After nucleation, the TPM oil can either be solidified by means of a radical polymerization reaction to obtain composite particles ( Fig. 1 ), or trivially dissolved in ethanol to recover the PS seeds (the importance of this step will be explained later). The composite colloids resulting from the polymerization of TPM now comprise two different polymers: a highly cross-linked silsesquioxanes (polymerized TPM), and a linear polymer (PS). In the figures presented in this paper, the two polymers are highlighted, respectively, in green and red. As the polymers are compartmentalized and have different chemistries, discrete portions of a particle can be selectively functionalized, polymerized or dissolved. 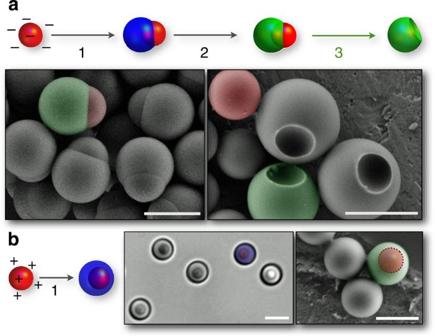Figure 1: Particles fabrication principle. Schematic diagram showing the synthetic steps involved in the preparation of particles with various types of protrusions and cavities. (a) Spherical PS seeds are encapsulated into polymerizable oil droplets via a seeded dispersion polymerization (step 1). Depending on the PS surface charge, the seeds can sit at the oil–water interface (negatively charged seeds, (a)) or be entirely engulfed in the oil (positively charged seeds, (b)). The oil is then hardened via a radical polymerization (step 2) to obtain particles with a protrusion. These colloids can be further processed to selectively dissolve the original seeds and obtain particles with well-defined cavities (step 3). False-colour scanning electron microscopy images highlight the seeds in red and the polymerized oil in green. A bright field microscopy image of unpolymerized composite particles is also shown in (b). Scale bars, 2 μm. Figure 1 , for example, shows how particles with well-defined spherical cavities are fabricated by selectively dissolving the original PS seed. In practice, this can be realized by washing the composite colloids in pure toluene, which rapidly dissolves the PS leaving the cross-linked polymer unaffected. Figure 1: Particles fabrication principle. Schematic diagram showing the synthetic steps involved in the preparation of particles with various types of protrusions and cavities. ( a ) Spherical PS seeds are encapsulated into polymerizable oil droplets via a seeded dispersion polymerization (step 1). Depending on the PS surface charge, the seeds can sit at the oil–water interface (negatively charged seeds, ( a )) or be entirely engulfed in the oil (positively charged seeds, ( b )). The oil is then hardened via a radical polymerization (step 2) to obtain particles with a protrusion. These colloids can be further processed to selectively dissolve the original seeds and obtain particles with well-defined cavities (step 3). False-colour scanning electron microscopy images highlight the seeds in red and the polymerized oil in green. A bright field microscopy image of unpolymerized composite particles is also shown in ( b ). Scale bars, 2 μm. Full size image Reshaping colloids If, instead of polymerizing the oil phase, we liquify the solid PS phase by allowing the seeds to absorb a small amount of toluene, an entirely new family of particle shapes can be generated. The liquified PS seeds do not mix with the TPM oil. However, because they are now liquid, surface tension gradually deform them from spheres to concave caps ( Fig. 2 ). The equilibrium shape of the whole multiphase particle will depend on the amount of toluene added, which in turn sets the contact angles between the three liquid phases: water, TPM oil and toluene-swollen PS [22] . We call this step deformation. 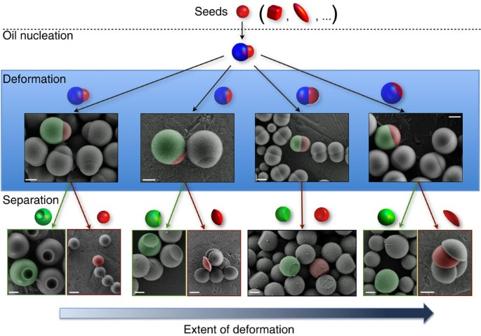Figure 2: Zoology of anisotropic particles. Our synthetic scheme involves three distinct steps. Nucleation: droplets of a polymerizable oil (TPM) are nucleated on preexisting PS seeds. Deformation: the addition of toluene causes the PS seeds to liquify and whole particles to deform under surface tension forces. The desired morphology is fixed by dripping of the toluene and polymerizing the oil. Separation: after polymerization, the newly shaped particles are comprised of two compartmentalized polymers: PS (red) and polymerized TPM (green). Each polymer can be selectively dissolved, effectively allowing us to split the composite particle into complementary pieces. Scale bars, 1 μm. Figure 2: Zoology of anisotropic particles. Our synthetic scheme involves three distinct steps. Nucleation: droplets of a polymerizable oil (TPM) are nucleated on preexisting PS seeds. Deformation: the addition of toluene causes the PS seeds to liquify and whole particles to deform under surface tension forces. The desired morphology is fixed by dripping of the toluene and polymerizing the oil. Separation: after polymerization, the newly shaped particles are comprised of two compartmentalized polymers: PS (red) and polymerized TPM (green). Each polymer can be selectively dissolved, effectively allowing us to split the composite particle into complementary pieces. Scale bars, 1 μm. Full size image Because of the slow rate at which this deformation occurs, the intermediate out-of-equilibrium shapes can be followed by optical microscopy and fixed at will by stripping the toluene off and allowing the PS to return to a solid state. Separation into shape-complementary colloids From these newly shaped particles, a second generation of anisotropic and shape-complementary colloids is obtained by selectively dissolving one polymer or the other. In particular, the polymerized TPM part is recovered by washing the particles in toluene whereas the PS is isolated by washing the TPM oil off in ethanol before its polymerization. We call this last step separation as it effectively results in the subdivision of the composite particle into its two constituent polymers ( Fig. 2 ). Multi-lobe colloids By varying the experimental conditions during the nucleation step (see Methods section), multiple oil droplets can be controllably grown on the same seed to yield dumbbells or particles with multiple protrusions. As illustrated in Fig. 3 , this further extends the number of shapes that can be fabricated using our method. Overall, we were able to obtain bulk quantities of monodispersed colloids shaped like disks, bowls, lentils and dumbbells along with particles with well-defined cavities, flats and protrusions. 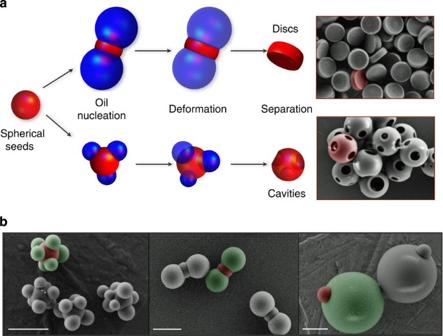Figure 3: Multiple cavities. (a) Depending on the experimental conditions, the oil (shown in blue) can nucleate on the seeds (shown in red) forming a single lobe, two opposite lobes or multiple lobes. This gives access to particle morphologies that further extend the one shown inFig. 2. (b) Scanning electron microscopy images showing PS spheres (in red) featuring one, two or multiples TPM lobes (in green). Scale bars, 2 μm. Figure 3: Multiple cavities. ( a ) Depending on the experimental conditions, the oil (shown in blue) can nucleate on the seeds (shown in red) forming a single lobe, two opposite lobes or multiple lobes. This gives access to particle morphologies that further extend the one shown in Fig. 2 . ( b ) Scanning electron microscopy images showing PS spheres (in red) featuring one, two or multiples TPM lobes (in green). Scale bars, 2 μm. Full size image Anisotropic functionalization The different nature of our bi-material particles also opens new avenues to fabricating Janus or patchy colloids in bulk amounts. Silane chemistry, for example, can be selectively performed on the organosilica polymer leaving the PS unaffected, whereas hydrophobic molecules, such as fluorescent dyes, can be preferentially absorbed and concentrated in the PS phase and remain physically or chemically trapped here. 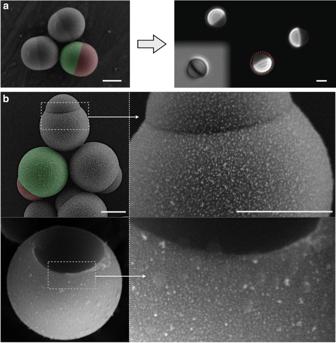Figure 4: Particles functionalization. To functionalize our particles, we can either exploit the different chemical reactivity of PS and TPM or use one polymer as a sacrificial protective layer. In (a), we show Janus-like colloids that were fabricated in bulk by trapping and locking dye molecules into the PS phase via a two-step swelling and polymerization process. The picture shows an scanning electron microscopy (SEM) image of the particles on the left side and a fluorescence optical microscopy image of the same particles on the right side (bright field view in the insert). In (b), SEM images show the steps involved in the synthesis of colloids with a partially coated surface. First, gold nanoparticles are homogeneously adsorbed onto a composite particle, and then the one part of the particle is selectively dissolved to reveal an uncoated surface. Scale bars, 1 μm. Figure 4 shows fluorescent Janus colloids that were prepared by first swelling the PS hemisphere of TPM–PS composite particles with a polymerizable fluorophore (NBD-MAEM [23] ), followed by a locking polymerization reaction to fix the fluorescent dye inside the particles. Alternatively, TPM-soluble molecules can be added to the oil before its polymerization and chemically bonded via silane chemistry. This was tested by adding rhodamine-B-isothiocyanate dye coupled with 3-aminopropyltriethoxysilane (RITC-APS) to a suspension of biphasic particles before the polymerization of the TPM phase. The fluorescent dye covalently binds only to the TPM phase as a result of a condensation reaction between the APS and TPM silane moieties. Figure 4: Particles functionalization. To functionalize our particles, we can either exploit the different chemical reactivity of PS and TPM or use one polymer as a sacrificial protective layer. In ( a ), we show Janus-like colloids that were fabricated in bulk by trapping and locking dye molecules into the PS phase via a two-step swelling and polymerization process. The picture shows an scanning electron microscopy (SEM) image of the particles on the left side and a fluorescence optical microscopy image of the same particles on the right side (bright field view in the insert). In ( b ), SEM images show the steps involved in the synthesis of colloids with a partially coated surface. First, gold nanoparticles are homogeneously adsorbed onto a composite particle, and then the one part of the particle is selectively dissolved to reveal an uncoated surface. Scale bars, 1 μm. Full size image Another powerful strategy for functionalizing only part of the particle’s surface and realize more complex patchy colloids is to employ one of the two polymer species as a sacrificial protective layer. We demonstrate this concept in Fig. 4 where composite TPM–PS particles were first homogeneously coated by gold nanoparticles and then washed in toluene to remove the PS and expose an uncoated TPM surface (see more details in the Methods section). Gold-coated anisotropic particles, in particular, are of interest not only in self-assembly [24] , [9] but also in biomedical applications as gold offers a versatile substrate for further functionalization, including fluorescent markers, DNA and other biomolecules [25] . This coating procedure is not limited to gold nanoparticles and can be further extended to include other inorganic colloids, such as iron oxides. In the Supplementary Material , for example, we show how we also used magnetite nanoparticles to prepare magnetizable building blocks that can be remotely manipulated with the use of external fields ( Supplementary Movie S1 and Supplementary Figs S3, S4 ). Self-assembly Another important feature of our method is the ability to produce colloidal building blocks with perfect shape complementarity. In a previous work [3] , we showed how shapes can be exploited to drive selective lock-and-key binding between colloids, thus realizing a simple mechanism of particle recognition and binding. This mechanism, however, required independently fabricating sets of complementary building blocks whose matching geometries were generally obtained via a lengthy trial-and-error iterative process. With our new approach, we greatly simplify the synthesis of such colloidal particles, as the complementary pieces are now simultaneously generated by an effective subdivision of composite particles ( Fig. 2 ). This is shown in Supplementary Fig. S2 where we use depletion forces to organize the particles into architectures, which are determined by the geometry of the constituent building blocks. Finally, we point to the universality of the synthetic principle, by demonstrating its applicability to a variety of seeds other than spherical PS. By using differently shaped seeds, in fact, we can generate an even larger particle library featuring shapes that can be designed a priori by treating the synthesis as a simple wetting problem. In Fig. 5a , for example, the oil was nucleated in the presence of elongated seeds obtained by stretching regular sulphonated PS spheres [26] . This resulted in spherical particles with identical ellipsoidal dimples. Similarly, we can use cubic seeds of haematite to produce particles with cubic cavities as illustrated in Fig. 5b . 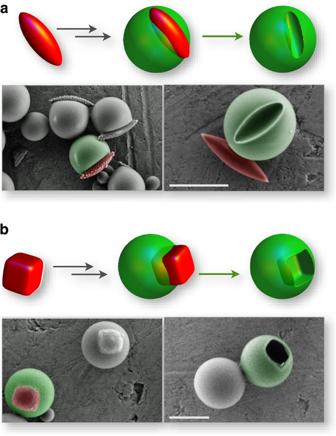Figure 5: Shaping cavities. Seeds with various shapes and compositions were used to fabricate particles with well-defined cavities. (a) Shows particles with ellipsoidal dimples that were obtained from elongated PS seeds. (b) Shows particles with cubic cavities shaped by cubic seeds of haematite. Scale bars, 2 μm. Figure 5: Shaping cavities. Seeds with various shapes and compositions were used to fabricate particles with well-defined cavities. ( a ) Shows particles with ellipsoidal dimples that were obtained from elongated PS seeds. ( b ) Shows particles with cubic cavities shaped by cubic seeds of haematite. Scale bars, 2 μm. Full size image In summary, we have developed a new and general synthetic roadmap for fabricating colloidal particles featuring tunable shapes and tailored surface properties. Our method seamlessly combines the design freedom of a multistep synthesis with the scalability of a bulk process, yielding highly customizable colloidal building blocks that are of interest for studying self-assembling mechanisms as well as for technological applications. The particles prepared via the initial heterogeneous nucleation step, for example, can be designed to incorporate virtually any type of organic and inorganic seed into the oil, thus resulting into composite particles with active cores or protrusions [27] , [28] . The contact lens-like particles that we prepared via deformation of spherical PS colloids are expected to exhibit a novel phase behaviour [29] and because of their tunable size and convexity are also of potential interest as a source of building blocks for the assembly of microlens arrays [30] , [31] . The shape-complementary particle pairs obtained via the separation step feature tunable complex geometries that are excellent tools to explore self-assembly mechanisms via lock-and-key interactions [32] . Finally, by exploiting the compartmentalization and the different chemistry of the polymers forming our our biphasic particles, we have demonstrated that our synthetic method can also stretch to the preparation of patchy and Janus colloids. Heterogeneous nucleation of TPM droplets In a typical experiment, 6 ml of TPM (≥98% from Sigma-Aldrich) was hydrolysed in 60 ml of deionized water by vigorous stirring for about 5 h. Next, 6 ml of this solution was rapidly mixed with 8 ml of an aqueous suspension containing 3 μl of NH 3 28% and 100 μl of a stock seeds suspension (1.4 μm negatively charged PS spheres from Life Technologies, Sulfate Latex, 8% w/v). Occasionally, various other seeds were used: 1 and 1.2 μm negatively charged PS spheres (Life Technologies, Sulfate Latex, 8% w/v), 1.4 μm positively charged PS spheres (Life Technologies, Amidine Latex, 8% w/v), negatively charged PS rods (kindly provided by the Solomon group and prepared following the method described by Ho et al . [33] ) and haematite cubes (synthesized following the method described by Sugimoto [34] ). The mixture was left undisturbed for up to 30 min to allow the TPM droplets to nucleate and grow on the seeds. Occasionally, the addition of TPM was repeated a few times to obtain the desired particles size. The whole process of nucleation and growth was carefully monitored by optical microscopy at regular intervals using a Nikon inverse microscope equipped with a × 100 Nikon oil objective and a CoolSNAP EZ Photometrics CCD camera. At low seed concentration of ~0.017% (corresponding to 100 μl of the stock 8% w/v seeds suspension added to 30 ml of water), the TPM nucleates almost exclusively on the PS seeds forming a single droplet. However, when the seed concentration is raised to ~0.044% (250 μl of the stock suspension), the particle morphology changes dramatically and monodisperse dumbbells, consisting in a central PS sphere and two opposite TPM lobes, are obtained ( Supplementary Fig. S1 ). Very small TPM droplets are often observed as a result of secondary (homogeneous) nucleation but are easily separated via a few sedimentation and resuspension cycles. To test the applicability of our method to nano-scale seeds, we also preformed a few experiments using 100-nm PS spheres as follows: 6 μl of NH 3 28% and 200 μl of a 15 wt PS suspension were added under stirring to 10 μl of water followed by 600 μl of TPM. The mixture was left under stirring for 1 h and polymerized as described above. Similarly, iron oxide nanorods were used to nucleate 200 nm TPM droplets. The resulting nano-sized colloids are shown in the Supplementary Fig. S5 . Deformation and fixation of the PS phase After the nucleation of the TPM droplets, the spherical PS seeds were plasticized and progressively deformed by adding small amounts of toluene (typically in the order of 100 μl of toluene per 30 ml suspension). The suspensions were then left under mild stirring for a few hours and the morphological changes were carefully followed by optical microscopy. Various intermediate non-equilibrium structures ( Fig. 2 ) were fixed by stirring the suspension at 80 °C in an open container and allowing the toluene to evaporate and the PS phase to re-solidify. Dissolution of the TPM phase The newly shaped PS particles were isolated by washing the composite particles in ethanol to dissolve the unpolymerized TPM. The so recovered PS particles were resuspended in deionized water. Polymerization of the TPM phase To polymerize the TPM phase, 0.5 mg of 2,2′-azo-bis-isobutyrylnitrile (AIBN, Sigma-Aldrich) were added to the suspension and the mixture heated at 80 °C for 3 h. After the reaction, the particles were cleaned by sedimentation and resuspension in pure water. Dissolution of the PS phase To dissolve the PS seeds and obtain colloids with cavities, the polymerized particles were first resuspended in anhydrous ethanol and then washed in pure toluene. When the PS seeds were completely dissolved, the remaining TPM particles were transferred back to ethanol and finally to pure water. Dissolution of the Haematite phase Haematite cubes were chemically etched off the composite particles by adding concentrated hydrochloric acid (HCl 37%wt, Acros) directly into the particle suspension to a final HCl concentration of 5 M. After typically 12 h, the haematite fully dissolved and the remaining polymer particles were washed several times in deionized water until a neutral pH was reached. Gold and magnetic coating Inorganic nanoparticles were bound onto our composite colloids via amine-group linkages mediated by a silane-coupling agent (3-(ethoxydimethylsilyl)propylamine, 97%, Sigma-Aldrich). The coupling agent was anchored on polymerized TPM–PS particles via a condensation reaction as follows: 5 μl of 3-(ethoxydimethylsilyl)propylamine and 5 μl of tetramethylammonium hydroxide (TMAH, 25% in water, Acros) were added, under stirring, to a 20 ml suspension of particles in anhydrous ethanol and left to react overnight. The modified particles were washed twice in ethanol to remove unreacted silanes and then resuspended in deionized water. The inversion in the measured zeta potential from −7 to +30 mV (measured at neutral pH) confirmed the successful surface modification. Next, this aqueous suspension was concentrated by reducing its volume to 1 ml and then rapidly injected into a 10 ml aqueous suspension of nanoparticles. The mixture was left under stirring for 10 min before washing the excess of nanoparticles off via sedimentation and redispersion in pure water. Gold nanoparticles were prepared by reducing Au(III) (AuCl 3 trihydrate, 99.9%, Sigma-Aldrich) using sodium borohydride (NaBH 4 , ≥98%, Sigma-Aldrich). Briefly, 1 ml of NaBH 4 0.1 M was rapidly added to a 20 ml AuCl 3 0.1 mM solution kept under vigorous stirring. The formation of the gold sol is instantaneous and the resulting suspension was used without further purification. Magnetite (Fe 3 O 4 ) nanoparticles were prepared following the method described by Massart [35] . Assembly experiments Poly(ethylene oxide) (PEO, Acros Organics) with a molecular weight of 600 000 was used as depletant to drive the particle’s self-assembly. Depending on the colloidal system, various concentrations of PEO were used (typically between 0.3 and 1.2 g l −1 ). In all the experiments, the ionic strength was fixed at 5 mM NaCl. The assembly experiments were performed confining the particle suspensions in sealed borosilicate glass capillary (inner dimensions 2.0 × 0.1 mm 2 , Vitrocom). How to cite this article: Sacanna, S. et al . Shaping colloids for self-assembly. Nat. Commun. 4:1688 doi:10.1038/ncomms2694 (2013).